Identification of the phytosphingosine metabolic pathway leading to odd-numbered fatty acids The long-chain base phytosphingosine is a component of sphingolipids and exists in yeast, plants and some mammalian tissues. Phytosphingosine is unique in that it possesses an additional hydroxyl group compared with other long-chain bases. However, its metabolism is unknown. Here we show that phytosphingosine is metabolized to odd-numbered fatty acids and is incorporated into glycerophospholipids both in yeast and mammalian cells. Disruption of the yeast gene encoding long-chain base 1-phosphate lyase, which catalyzes the committed step in the metabolism of phytosphingosine to glycerophospholipids, causes an ~40% reduction in the level of phosphatidylcholines that contain a C15 fatty acid. We also find that 2-hydroxypalmitic acid is an intermediate of the phytosphingosine metabolic pathway. Furthermore, we show that the yeast MPO1 gene, whose product belongs to a large, conserved protein family of unknown function, is involved in phytosphingosine metabolism. Our findings provide insights into fatty acid diversity and identify a pathway by which hydroxyl group-containing lipids are metabolized. Cell membranes contain thousands of lipid species, which have compositions specific to each organism, tissue, cell and organelle and become altered in response to environmental changes. Cell membranes with certain lipid compositions exhibit characteristic properties of fluidity, thickness, curvature and local crowding (lipid microdomain), affecting protein activities and cellular signalling. Maintenance of cell- or tissue-specific lipid composition is important for cellular activity, and its deregulation leads to disorders. Fatty acids (FAs), the hydrophobic backbones of most lipid classes, are diverse molecules differing in chain-length, degree of saturation and modification state, for instance, hydroxylation. Most cellular FAs contain even-numbered chain-lengths. However, odd-numbered FAs also exist, albeit at much lesser levels compared with even-numbered FAs [1] , [2] , [3] , [4] . Sphingolipids are one of the major lipid classes in eukaryotes. Their roles are not restricted to building blocks of plasma membrane but also include cell adhesion, recognition of viruses and bacterial toxins, skin barrier formation, neural functions, apoptosis and glucose metabolism [5] , [6] , [7] , [8] , [9] . Furthermore, the sphingolipid metabolite sphingosine 1-phosphate (S1P) functions as a lipid mediator that regulates various cellular responses, such as egress of T cells from the thymus and secondary lymphoid tissues and vascular stabilization, by binding to one of the five S1P receptors (S1P 1–5 ) [6] , [10] . Its function in the immune system has already been applied clinically as a therapeutic agent for multiple sclerosis [11] . The hydrophobic backbone of the sphingolipid ceramide (Cer) is composed of a long-chain base (LCB) and a FA connected by an amide bond [6] . The major LCB in mammals is a trans -double bond-containing sphingosine, which is a precursor of S1P. Sphingosine/LCB is phosphorylated by sphingosine/LCB kinases to produce S1P/LCB 1-phosphate (LCBP). The saturated LCB dihydrosphingosine (DHS) also exists throughout the body, although the levels of DHS are less abundant than those of sphingosine [6] . Phytosphingosine (PHS), which contains a hydroxyl group at the C4 position, is localized to specific tissues such as the skin and small intestine [7] , [12] , [13] , [14] . PHS is a major LCB in yeast, and it also exists in plants [15] . In addition to the function of S1P/LCBP as a lipid mediator, S1P/LCBP also plays an important role as an intermediate in the sphingolipid-to-glycerophospholipid metabolic pathway [16] . This metabolic pathway is conserved in eukaryotes from yeast to humans, indicating its much older origin than the function of S1P/LCBP as a lipid mediator. We recently identified the complete metabolic pathway of S1P. S1P is metabolized to palmitoyl-CoA via four reactions (cleavage, oxidation, CoA addition and saturation) and incorporated into glycerophospholipids [17] , [18] , [19] . DHS is also metabolized to glycerophospholipids after phosphorylation through a pathway that is essentially same as the S1P metabolic pathway, but without the saturation step [17] ( Fig. 1a ). However, current knowledge about the metabolism of PHS is severely lacking. For example, it is even unknown whether PHS is metabolized to glycerophospholipids. If it is metabolized to glycerophospholipids, it still remains unclear whether PHS is incorporated into glycerophospholipids as FA or 2-hydroxy FA. 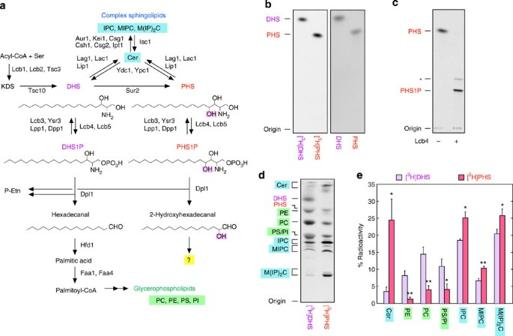Figure 1: PHS is metabolized to both sphingolipids and glycerophospholipids. (a) Shown are pathways of sphingolipid biosynthesis and degradation as well as the enzymes involved in each step. In thede novosphingolipid biosynthetic pathway, acyl-CoA and serine are condensed to 3-ketodihydrosphingosine (KDS), which is then reduced to DHS. DHS or its hydroxylated product PHS is acylated to generate Cer. Cer is converted to complex sphingolipids (IPC, MIPC and M(IP2)C) by receiving phosphoinositol, mannose and second phosphoinositol, successively. Some DHS and PHS are phosphorylated by LCB kinase to DHS1P and PHS1P, respectively. These LCBPs are either dephosphorylated by LCBP phosphatases to LCBs or cleaved between the 2- and 3-positions by the LCBP lyase Dpl1, generating fatty aldehydes (hexadecanal and 2-hydroxyhexadecanal, respectively) and phosphoethanolamine (P-Etn). Hexadecanal is converted to glycerophospholipids (PC, phosphatidylethanolamine, phosphatidylinositol and phosphatidylserine) via palmitic acid and palmitoyl-CoA. However, the metabolism of 2-hydroxyhexadecanal is unclear and is the subject of this study. (b) [11,12-3H]PHS prepared in this study and [4,5-3H]DHS purchased from American Radiolabeled Chemicals, each at 0.1 μCi, together with cold DHS and PHS, each at 10 nmol, were separated by normal-phase TLC with chloroform/methanol/4.2 N ammonia (9:7:2, v/v). Labelled and cold lipids were detected by autoradiography (left panel) and ninhydrin staining (right panel), respectively. (c) [3H]PHS (8 nCi) was incubated with or without purified 3xFLAG-Lcb4 (250 ng) in the presence of 5 mM ATP at 37 °C for 1 h. Lipids were extracted, separated by normal-phase TLC with chloroform/methanol/4.2 N ammonia (9:7:2, v/v) and detected by autoradiography. The asterisk indicates an undetermined PHS1P derivative. (d) BY4741 (wild-type) cells were labelled with 0.1 μCi [3H]DHS or [3H]PHS at 30 °C for 3 h. Lipids were extracted, separated by normal-phase TLC with chloroform/methanol/4.2 N ammonia (9:7:2, v/v) and detected by autoradiography. (e) The radioactivity associated with each lipid indwas quantified, and the data are expressed as the mean±s.d. relative to the radioactivity in the total lipids from three independent experiments. Statistically significant differences are indicated (Student’st-test; *P<0.05; **P<0.01). Figure 1: PHS is metabolized to both sphingolipids and glycerophospholipids. ( a ) Shown are pathways of sphingolipid biosynthesis and degradation as well as the enzymes involved in each step. In the de novo sphingolipid biosynthetic pathway, acyl-CoA and serine are condensed to 3-ketodihydrosphingosine (KDS), which is then reduced to DHS. DHS or its hydroxylated product PHS is acylated to generate Cer. Cer is converted to complex sphingolipids (IPC, MIPC and M(IP 2 )C) by receiving phosphoinositol, mannose and second phosphoinositol, successively. Some DHS and PHS are phosphorylated by LCB kinase to DHS1P and PHS1P, respectively. These LCBPs are either dephosphorylated by LCBP phosphatases to LCBs or cleaved between the 2- and 3-positions by the LCBP lyase Dpl1, generating fatty aldehydes (hexadecanal and 2-hydroxyhexadecanal, respectively) and phosphoethanolamine (P-Etn). Hexadecanal is converted to glycerophospholipids (PC, phosphatidylethanolamine, phosphatidylinositol and phosphatidylserine) via palmitic acid and palmitoyl-CoA. However, the metabolism of 2-hydroxyhexadecanal is unclear and is the subject of this study. ( b ) [11,12- 3 H]PHS prepared in this study and [4,5- 3 H]DHS purchased from American Radiolabeled Chemicals, each at 0.1 μCi, together with cold DHS and PHS, each at 10 nmol, were separated by normal-phase TLC with chloroform/methanol/4.2 N ammonia (9:7:2, v/v). Labelled and cold lipids were detected by autoradiography (left panel) and ninhydrin staining (right panel), respectively. ( c ) [ 3 H]PHS (8 nCi) was incubated with or without purified 3xFLAG-Lcb4 (250 ng) in the presence of 5 mM ATP at 37 °C for 1 h. Lipids were extracted, separated by normal-phase TLC with chloroform/methanol/4.2 N ammonia (9:7:2, v/v) and detected by autoradiography. The asterisk indicates an undetermined PHS1P derivative. ( d ) BY4741 (wild-type) cells were labelled with 0.1 μCi [ 3 H]DHS or [ 3 H]PHS at 30 °C for 3 h. Lipids were extracted, separated by normal-phase TLC with chloroform/methanol/4.2 N ammonia (9:7:2, v/v) and detected by autoradiography. ( e ) The radioactivity associated with each lipid in d was quantified, and the data are expressed as the mean±s.d. relative to the radioactivity in the total lipids from three independent experiments. Statistically significant differences are indicated (Student’s t -test; * P <0.05; ** P <0.01). Full size image Several organisms, including bacteria, fungi, plants and animals, possess 2-hydroxy FAs [20] . In mammals, 2-hydroxy FAs exist in specific tissues such as the epidermis, small intestine and in myelin [7] , [21] , [22] . An additional hydroxyl group in 2-hydroxy FA as well as in PHS may confer the unique ability to strongly interact with other lipids and proteins via an extra hydrogen bond. In myelin, 2-hydroxy FAs are enriched in the glycosphingolipids galactosylceramide and sulfatide, and may have important functions in the firm stacking of multiple lipid layers. Mutations in the gene encoding FA 2-hydroxylase ( FA2H ) cause hereditary spastic paraplegia, a neuronal disorder [23] . In the stratum corneum of the epidermis, multiple lipid lamellae act as a permeability barrier. Ceramides containing 2-hydroxy FAs and PHS are particularly abundant in the lipid lamellae [7] , and their hydroxyl groups may also strengthen the interaction between lipid layers. Although the hydroxyl group confers this particular property to lipids, its presence renders their metabolism complex. As 2-hydroxy FAs are only incorporated into sphingolipids and are resistant to β-oxidation, 2-hydroxy FAs must be converted to other metabolizable compounds for utilization in other lipid species or for removal. However, as with PHS metabolism, the metabolic pathway of 2-hydroxy FAs is largely unknown. In the present study, we prepared radiolabelled PHS and first examined its metabolism using yeast as a model organism, as PHS is a major LCB in yeast [24] . We then expanded the analyses to mammalian cells. We found that PHS was metabolized to sphingolipids and glycerophospholipids as other LCBs. Interestingly, PHS was metabolized to odd-numbered FAs in glycerophospholipids via the intermediate 2-hydroxypalmitic acid. Deletion of the yeast LCBP lyase gene ( DPL1 ), which is responsible for the first step of LCBP metabolism, caused a reduction in the levels of the C15 phosphatidylcholine (PC) species to ~40% of the control, indicating that PHS is the major source of odd-numbered FAs in yeast. Furthermore, we identified that the yeast MPO1 (Metabolism of PHS to Odd-numbered FA) gene is involved in PHS metabolism. Mpo1 belongs to the large protein family DUF962 (DUF: Domain of Unknown Function), whose function presently is completely unknown. We speculate that Mpo1 acts as an α-oxidase of 2-hydroxyacyl-CoA. Through the pathway revealed here, PHS and 2-hydroxy FAs are converted to metabolizable, saturated FAs (odd-numbered FAs). As deregulated accumulation of biomolecules often leads to cellular dysfunction or disorder, our newly identified PHS metabolic pathway may also be important for the maintenance of proper cellular functions. PHS is metabolized to odd-numbered FAs The metabolism of PHS is currently unknown mainly due to the lack of commercially available radioactive PHS. Therefore, we prepared radiolabelled PHS ([11,12- 3 H]PHS) from [9,10- 3 H]palmitic acid by metabolic conversion in yeast, followed by purification. The prepared [ 3 H]PHS presented as a single band that migrated to a position identical to a cold PHS standard on thin-layer chromatography (TLC; Fig. 1b ), suggesting that our [ 3 H]PHS was highly pure. Furthermore, all [ 3 H]PHS was converted to PHS 1-phosphate (PHS1P) upon incubation with LCB kinase Lcb4 ( Fig. 1c ), confirming its identity and purity. We observed additional lipid products in addition to PHS1P following Lcb4 treatment ( Fig. 1c , asterisk). Similar lipids were reported in a previous study [25] , where the authors concluded that these lipids were generated during the TLC separation. To examine the metabolism of PHS, wild-type yeast cells were labelled with [ 3 H]PHS or [ 3 H]DHS, for comparison, and their metabolites were separated by TLC ( Fig. 1d ). Consistent with a previous report [17] ( Fig. 1a ), DHS was metabolized to sphingolipids (Cer inositol phosphorylceramide (IPC), mannosylinositol phosphorylceramide (MIPC) and mannosyldiinositol phosphorylceramide (M(IP) 2 C)) and glycerophospholipids (PC, phosphatidylethanolamine (PE), phosphatidylserine (PS) and phosphatidylinositol (PI)). Similar to DHS metabolism, PHS was metabolized to both sphingolipids and glycerophospholipids, but with the metabolic flow to sphingolipids being predominant ( Fig. 1e ). To characterize the FA composition of these glycerophospholipids, [ 3 H]DHS/[ 3 H]PHS metabolites were subjected to mild saponification that hydrolyzes ester-linked FAs from glycerophospholipids without hydrolysis of amide-linked FAs from sphingolipids. The liberated FAs were esterified to FA methyl-esters (FAMEs) and analyzed by reverse-phase TLC ( Fig. 2a ) along with standard FAMEs ( Supplementary Fig. 1 ). A portion of the FAME mixture was also treated with KIO 4 -KMnO 4 before TLC analysis to identify saturated and unsaturated FAs ( Fig. 2b ). The KMnO 4 -KIO 4 treatment oxidatively cleaves a double bond, thus fragmenting unsaturated FAs; consequently, the spot corresponding to the unsaturated FA disappears on the TLC. DHS was metabolized to palmitoyl-CoA (C16:0) and palmitoleoyl-CoA (C16:1), the latter of which was formed by Δ9 desaturase-catalyzed reaction of the former, and subsequently to glycerophospholipids. On the other hand, PHS was incorporated into glycerophospholipids as odd-numbered FAs (C15:0 and, to a lesser extent, C15:1; Fig. 2a,b ). 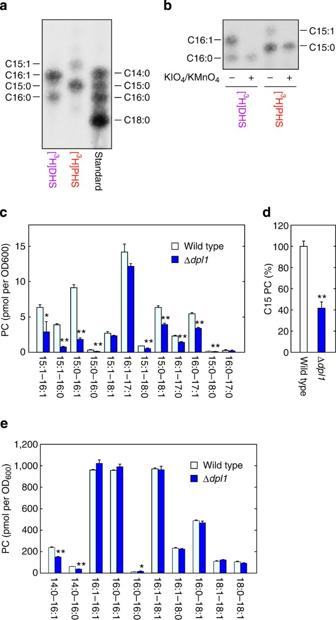Figure 2: PHS is metabolized to odd-numbered FAs in yeast. (a,b) BY4741 (wild-type) cells were labelled with 0.2 μCi [3H]DHS or [3H]PHS at 30 °C for 3 h. Lipids were extracted, treated with alkaline solution and separated by normal-phase TLC with chloroform/methanol/4.2 N ammonia (9:7:2, v/v). FAs were scraped from TLC, eluted from TLC silica and methyl-esterified. (a) FAMEs were separated by reverse-phase TLC with chloroform/methanol/water (5:15:1, v/v) and detected by autoradiography. The standard containing C14:0, C15:0, C16:0 and C18:0 FAMEs was a mixture of FA elongation products prepared inSupplementary Fig. 1. (b) FAMEs were treated with/without aqueous KMnO4/KIO4, extracted with hexane and separated by reverse-phase TLC with chloroform/methanol/water (5:15:1, v/v). (c–e) BY4741 and 3653 (Δdpl1) cells were grown in SC medium at 30 °C. Lipids were extracted from these cells and separated by normal-phase TLC with chloroform/methanol/4.2 N ammonia (9:7:2, v/v). PC was collected from TLC plates, and its composition was analyzed by UPLC-MS with a Xevo G2 QTof LC/MS system. The data were analyzed with MassLynx software. (c,e) Each bar represents the amount of each PC species (c, odd-numbered PC;e, even-numbered PC) and the mean±s.d. from three independent experiments. (d) Values represent percent of the sum amounts of C15 PC species increlative to those in wild-type cells. Statistically significant differences are indicated (Student’st-test; *P<0.05, **P<0.01). Figure 2: PHS is metabolized to odd-numbered FAs in yeast. ( a , b ) BY4741 (wild-type) cells were labelled with 0.2 μCi [ 3 H]DHS or [ 3 H]PHS at 30 °C for 3 h. Lipids were extracted, treated with alkaline solution and separated by normal-phase TLC with chloroform/methanol/4.2 N ammonia (9:7:2, v/v). FAs were scraped from TLC, eluted from TLC silica and methyl-esterified. ( a ) FAMEs were separated by reverse-phase TLC with chloroform/methanol/water (5:15:1, v/v) and detected by autoradiography. The standard containing C14:0, C15:0, C16:0 and C18:0 FAMEs was a mixture of FA elongation products prepared in Supplementary Fig. 1 . ( b ) FAMEs were treated with/without aqueous KMnO 4 /KIO 4 , extracted with hexane and separated by reverse-phase TLC with chloroform/methanol/water (5:15:1, v/v). ( c – e ) BY4741 and 3653 (Δ dpl1 ) cells were grown in SC medium at 30 °C. Lipids were extracted from these cells and separated by normal-phase TLC with chloroform/methanol/4.2 N ammonia (9:7:2, v/v). PC was collected from TLC plates, and its composition was analyzed by UPLC-MS with a Xevo G2 QTof LC/MS system. The data were analyzed with MassLynx software. ( c , e ) Each bar represents the amount of each PC species ( c , odd-numbered PC; e , even-numbered PC) and the mean±s.d. from three independent experiments. ( d ) Values represent percent of the sum amounts of C15 PC species in c relative to those in wild-type cells. Statistically significant differences are indicated (Student’s t -test; * P <0.05, ** P <0.01). Full size image The contribution of PHS-to-glycerophospholipid metabolism to cellular odd-numbered FA levels was examined by analyzing the most abundant glycerophospholipid, PC, in LCBP lyase-deficient yeast cells (Δ dpl1 ) using liquid chromatography–mass spectrometry. In Δ dpl1 cells lacking the PHS-to-glycerophospholipid metabolic pathway ( Fig. 1a ; see also Fig. 4a ), most C15 PC species were significantly reduced ( Fig. 2c ). Deletion of the DPL1 gene caused a reduction in total C15 PC levels to ~40% of wild-type levels ( Fig. 2d ). Some PC species with an elongated C17 FA were also decreased ( Fig. 2c ), whereas those with two even-numbered FAs were mostly unaffected ( Fig. 2e ). Similar results were obtained when the deletion mutant of the SUR2 gene, which encodes the DHS C4-hydroxylase producing PHS from DHS, was analysed ( Supplementary Fig. 2 ). Figure 4: Pentadecanoic acid and 2-hydroxypalmitic acid are accumulated in the medium of acyl-CoA synthetase-deficient cells. 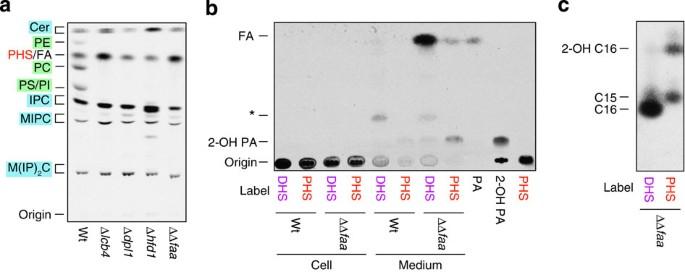Figure 4: Pentadecanoic acid and 2-hydroxypalmitic acid are accumulated in the medium of acyl-CoA synthetase-deficient cells. (a) BY4741 (wild-type; wt), 2427 (Δlcb4), 3653 (Δdpl1), 6550 (Δhfd1) and AOY13 (Δfaa1Δfaa4; ΔΔfaa) cells were incubated with 0.2 μCi [3H]PHS at 30 °C for 3 h. Lipids were extracted and separated by normal-phase TLC with chloroform/methanol/4.2 N ammonia (9:7:2, v/v). (b) BY4741 and AOY13 cells were incubated with 0.2 μCi [3H]DHS/[3H]PHS at 30 °C for 3 h. Lipids were extracted from the cell pellets and cell culture medium, separated by normal-phase TLC with hexane/diethyl ether/acetic acid (30:70:1, v/v) and detected by autoradiography. Asterisk indicates unidentified lipid. 2-Hydroxypalmitic acid (2-OH PA) was prepared by incubating [3H]PHS1P with purified S1P lyase and fatty aldehyde dehydrogenase. PA, palmitic acid. (c) AOY13 cells were incubated with 0.4 μCi [3H]DHS/[3H]PHS at 30 °C for 3 h. Lipids were extracted from culture medium, saponified and methyl-esterified. The resulting FAMEs were separated by reverse-phase TLC. ( a ) BY4741 (wild-type; wt), 2427 (Δ lcb4 ), 3653 (Δ dpl1 ), 6550 (Δ hfd1 ) and AOY13 (Δ faa1 Δ faa4 ; ΔΔ faa ) cells were incubated with 0.2 μCi [ 3 H]PHS at 30 °C for 3 h. Lipids were extracted and separated by normal-phase TLC with chloroform/methanol/4.2 N ammonia (9:7:2, v/v). ( b ) BY4741 and AOY13 cells were incubated with 0.2 μCi [ 3 H]DHS/[ 3 H]PHS at 30 °C for 3 h. Lipids were extracted from the cell pellets and cell culture medium, separated by normal-phase TLC with hexane/diethyl ether/acetic acid (30:70:1, v/v) and detected by autoradiography. Asterisk indicates unidentified lipid. 2-Hydroxypalmitic acid (2-OH PA) was prepared by incubating [ 3 H]PHS1P with purified S1P lyase and fatty aldehyde dehydrogenase. PA, palmitic acid. ( c ) AOY13 cells were incubated with 0.4 μCi [ 3 H]DHS/[ 3 H]PHS at 30 °C for 3 h. Lipids were extracted from culture medium, saponified and methyl-esterified. The resulting FAMEs were separated by reverse-phase TLC. Full size image When the pAN9 plasmid, which encoded the 3xFLAG-tagged DPL1 gene under the control of the GAPDH promoter, was introduced into the Δ dpl1 cells, C15 and C17 PC levels increased greatly, even when compared with the wild-type control ( Supplementary Fig. 3 ). Furthermore, addition of PHS to the culture medium caused a large increase in odd-numbered PCs ( Supplementary Fig. 4 ). Levels of some even-numbered PCs were also slightly altered by exogenous PHS. In summary, PHS is metabolized to odd-numbered FAs, and PHS appears to be a major source of odd-numbered FAs in yeast. LCBP lyase is a key determinant of LCB/LCBP metabolism The metabolism of PHS to glycerophospholipids was less efficient than that of DHS ( Fig. 1d ). However, it is unclear what determines LCB/LCBP metabolism. After LCBs are converted to LCBPs by LCB kinases, LCBPs are degraded via one of two reactions: cleavage by LCBP lyase to fatty aldehydes and phosphoethanolamine and dephosphorylation by LCBP phosphatases to LCBs [6] ( Fig. 1a ). Fatty aldehydes produced by LCBP lyase are metabolized to glycerophospholipids, whereas LCBs generated by LCBP phosphatases are recycled back to sphingolipids [6] . The yeast LCB kinases are reported to phosphorylate DHS and PHS with similar efficiencies [25] ; however, little is known about the relative activity of LCBP lyase/phosphatase towards DHS 1-phosphate (DHS1P) and PHS1P. In vitro LCBP lyase/phosphatase assays were therefore performed on [ 32 P]DHS1P and [ 32 P]PHS1P using membrane fractions, and the product [ 32 P]phosphoethanolamine/[ 32 P]phosphate was monitored by normal-phase TLC ( Fig. 3a ). Incubation of wild-type membranes with DHS1P produced almost equal amounts of phosphoethanolamine and phosphate (a 0.92:1 ratio), whereas phosphate was preferentially generated from PHS1P (a 0.45:1 ratio) (lines 3 and 4; see Fig. 3b for quantified data). Since Dpl1 is the sole LCBP lyase in yeast, the Δ dpl1 cell membranes did not produce phosphoethanolamine (lanes 5 and 6). However, deletion of the LCBP phosphatase Lcb3, the more predominant one of the two (Ysr3 being the other) [26] , was not sufficient to prevent the production of phosphate but reduced it with a concomitant increase of phosphoethanolamine (lanes 7 and 8). The lipid phosphate phosphatases Lpp1 and Dpp1 in yeast are known to exhibit broad specificity towards lipid phosphates [27] . Accordingly, DHS1P/PHS1P dephosphorylation was eliminated by using membranes of the Δ lcb3 Δ ysr3 Δ lpp1 Δ dpp1 quadruple deletion mutant (lanes 9 and 10). This result is consistent with our previous data indicating that membranes of the Δ lcb3 Δ lpp1 Δ dpp1 triple deletion mutant had no phosphatase activity towards DHS1P [28] . 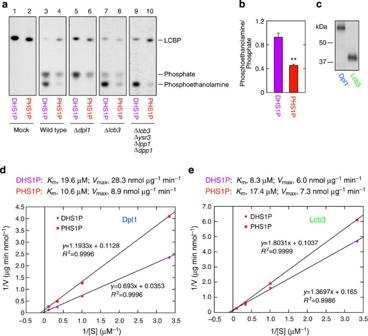Even under these phosphatase-null conditions, conversion of PHS1P to phosphoethanolamine was low (lane 10). Figure 3: PHS1P is more efficiently metabolized by LCBP phosphatases than LCBP lyase. (a,b) [32P]DHS1P/[32P]PHS1P (25 nCi, 0.5 μM) was incubated with buffer alone (mock) or a 5-μg total membrane fraction prepared from SEY6210 (wild-type), KHY13 (Δdpl1), KHY20 (Δlcb3) and KHY49 (Δlcb3Δysr3Δlpp1Δdpp1) cells at 37 °C for 10 min. (a) The reaction products were separated by normal-phase TLC with 1-butanol/acetic acid/water (2:1:1, v/v) and detected by autoradiography. (b) The radioactivity associated with [32P]phosphoethanolamine and [32P]phosphate in the wild-type membrane inawas quantified using a bioimaging analyzer BAS-2500. Values represent the mean±s.d. of the ratio of phosphoethanolamine to phosphate from three independent experiments. Statistically significant differences are indicated (Student’st-test; **P<0.01). (c) Total membrane fractions (0.8 μg) prepared from KHY80 (Δdpl1Δlcb3Δlpp1Δdpp1Δlcb4) cells harbouring the pAN9 (3xFLAG-DPL1) or pAN13 (3xFLAG-LCB3) plasmids were separated by SDS–polyacrylamide gel electrophoresis, followed by immunoblotting with anti-FLAG antibody. (d,e) Total membrane fractions (0.5 μg) prepared from KHY80/pAN9 (d) or KHY80/pAN13 (e) were incubated with 25 nCi32P-labelled DHS1P or PHS1P at 0.3, 1, 3 and 10 μM at 37 °C for 10 min. After termination of the reaction, reaction products were separated by normal-phase TLC, followed by detection and quantification using a bioimaging analyzer BAS-2500. The radioactivity associated with the reaction product phosphoethanolamine (d) or phosphate (e) was quantified. The 3xFLAG-Dpl1 and 3xFLAG-Lcb3 levels in the membrane fractions used were determined relative to the level of the 3xFLAG-maltose-binding protein standard and used for the calculation of the specific activity. We estimated that 1 μg of the total membrane fraction contained 3.2 ng of Dpl1 and 8.9 ng of Lcb3. The obtained values were expressed in a Lineweaver-Burk plot with a linear regression line.Rindicates the correlation coefficient. Figure 3: PHS1P is more efficiently metabolized by LCBP phosphatases than LCBP lyase. ( a , b ) [ 32 P]DHS1P/[ 32 P]PHS1P (25 nCi, 0.5 μM) was incubated with buffer alone (mock) or a 5-μg total membrane fraction prepared from SEY6210 (wild-type), KHY13 (Δ dpl1 ), KHY20 (Δ lcb3 ) and KHY49 (Δ lcb3 Δ ysr3 Δ lpp1 Δ dpp1 ) cells at 37 °C for 10 min. ( a ) The reaction products were separated by normal-phase TLC with 1-butanol/acetic acid/water (2:1:1, v/v) and detected by autoradiography. ( b ) The radioactivity associated with [ 32 P]phosphoethanolamine and [ 32 P]phosphate in the wild-type membrane in a was quantified using a bioimaging analyzer BAS-2500. Values represent the mean±s.d. of the ratio of phosphoethanolamine to phosphate from three independent experiments. Statistically significant differences are indicated (Student’s t -test; ** P <0.01). ( c ) Total membrane fractions (0.8 μg) prepared from KHY80 (Δ dpl1 Δ lcb3 Δ lpp1 Δ dpp1 Δ lcb4 ) cells harbouring the pAN9 ( 3xFLAG-DPL1 ) or pAN13 ( 3xFLAG-LCB3 ) plasmids were separated by SDS–polyacrylamide gel electrophoresis, followed by immunoblotting with anti-FLAG antibody. ( d , e ) Total membrane fractions (0.5 μg) prepared from KHY80/pAN9 ( d ) or KHY80/pAN13 ( e ) were incubated with 25 nCi 32 P-labelled DHS1P or PHS1P at 0.3, 1, 3 and 10 μM at 37 °C for 10 min. After termination of the reaction, reaction products were separated by normal-phase TLC, followed by detection and quantification using a bioimaging analyzer BAS-2500. The radioactivity associated with the reaction product phosphoethanolamine ( d ) or phosphate ( e ) was quantified. The 3xFLAG-Dpl1 and 3xFLAG-Lcb3 levels in the membrane fractions used were determined relative to the level of the 3xFLAG-maltose-binding protein standard and used for the calculation of the specific activity. We estimated that 1 μg of the total membrane fraction contained 3.2 ng of Dpl1 and 8.9 ng of Lcb3. The obtained values were expressed in a Lineweaver-Burk plot with a linear regression line. R indicates the correlation coefficient. Full size image The above results suggest that the differences in the metabolism of DHS and PHS ( Fig. 1d ) may be caused by different substrate preferences of the LCBP lyase Dpl1, but not of the LCBP phosphatases, towards DHS1P and PHS1P. To test this possibility, we next determined the kinetic parameters of Dpl1 and Lcb3 using cell membranes prepared from yeast cells lacking LCBP lyase and LCBP phosphatases but expressing 3xFLAG-tagged Dpl1 or Lcb3. Immunoblotting revealed that expression levels of 3xFLAG-Dpl1 and 3xFLAG-Lcb3 were equivalent ( Fig. 3c ). We determined the V max and K m values for Dpl1 to be 28.3 nmol μg −1 min −1 and 19.6 μM for DHS1P and 8.9 nmol μg −1 min −1 and 10.6 μM for PHS1P, respectively ( Fig. 3d ). Thus, the V max value of Dpl1 towards PHS1P is ~1/3 of that towards DHS1P, indicating that the activity of Dpl1 towards PHS1P was indeed low. On the other hand, the kinetic parameters of Lcb3 towards DHS1P and PHS1P were similar (DHS1P, 6.0 nmol μg −1 min −1 for V max and 8.3 μM for K m ; PHS1P, 7.3 nmol μg −1 min −1 for V max and 17.4 μM for K m ; Fig. 3e ). These results indicate that the activity of Dpl1 determines the efficiency of LCBP metabolism to glycerophospholipids. 2-Hydroxypalmitic acid is an intermediate in PHS metabolism We previously reported that DHS was metabolized to glycerophospholipids via DHS1P, hexadecanal, palmitic acid and palmitoyl-CoA [17] ( Fig. 1a ). The LCB kinase Lcb4, LCBP lyase Dpl1, fatty aldehyde dehydrogenase Hfd1 and acyl-CoA synthetases Faa1 and Faa4 are involved in each conversion step [17] ( Fig. 1a ). We next examined whether these enzymes were also involved in PHS metabolism. The PHS-to-glycerophospholipid conversion was completely abolished in Δ lcb4 , Δ dpl1 , Δ hfd1 and Δ faa1 Δ faa4 cells ( Fig. 4a ). Thus, the reactions catalyzed by the LCB kinase Lcb4, LCBP lyase Dpl1, fatty aldehyde dehydrogenase Hfd1 and acyl-CoA synthetases Faa1 and Faa4 are commonly required for DHS and PHS metabolism. Our results indicate that PHS is converted to PHS1P by Lcb4, to 2-hydroxyhexadecanal by Dpl1 and to 2-hydroxypalmitic acid by Hfd1. Consistent with the conclusion that 2-hydroxypalmitic acid is an intermediate of the PHS metabolic pathway, addition of 2-hydroxypalmitic acid to the culture medium caused an increase in odd-numbered PCs, as did addition of PHS ( Supplementary Fig. 4 ). To determine the reaction catalyzed by the acyl-CoA synthetases Faa1 and Faa4, we examined the FA species that accumulated in Δ faa1 Δ faa4 cells using normal-phase TLC and hexane/diethyl ether/acetic acid (30:70:1) as a resolving buffer. Although only small amounts of FAs were detected in the cell fraction of [ 3 H]PHS-labelled Δ faa1 Δ faa4 cells, FA and 2-hydroxy FA were observed in the medium ( Fig. 4b ). Methyl esterification and separation by reverse-phase TLC revealed that they were methyl esters of C15:0 FA (pentadecanoic acid) and 2-hydroxypalmitic acid ( Fig. 4c ). These FA intermediates were not observed in wild-type cells ( Fig. 4b ). When Δ faa1 Δ faa4 cells were labelled with [ 3 H]DHS, palmitic acid was found to accumulate in the medium ( Fig. 4b,c ), as expected from the metabolic pathway of DHS ( Fig. 1a ). MPO1 is involved in the metabolism of PHS The results described above indicate that PHS is metabolized to 2-hydroxypalmitic acid and then converted to pentadecanoic acid via α-oxidation. To identify a gene involved in α-oxidation of PHS metabolites, we performed bioinformatic analysis using a yeast database. As LCBP metabolism takes place in the endoplasmic reticulum (ER) [16] , we speculated that the corresponding gene encodes an ER protein. Therefore, we searched for genes encoding ER proteins in the yeast green fluorescent protein (GFP) fusion localization database ( http://yeastgfp.yeastgenome.org/ ) [29] and found 296 genes/open reading frames. Of these, the 13 genes with unknown functions were selected and their deletion mutants were subjected to the [ 3 H]PHS-labelling experiment. We found that one of these genes, termed MPO1 (Metabolism of PHS to Odd-numbered FA, open reading frame YGL010w ), exhibited a defect in the metabolism of PHS to glycerophospholipids when the gene was deleted ( Supplementary Fig. 5 ). Deletion of the MPO1 gene had no effect on DHS metabolism ( Fig. 5a ). These results indicate that the MPO1 gene is involved in a PHS-specific reaction, α-oxidation of PHS metabolites. Moreover, Δ mpo1 cells with [ 3 H]PHS accumulated 2-hydroxypalmitic acid in the medium ( Fig. 5b ). These results suggest that 2-hydroxypalmitic acid or its reversible metabolite is the substrate of Mpo1 and is released into the medium without accumulating in cells. 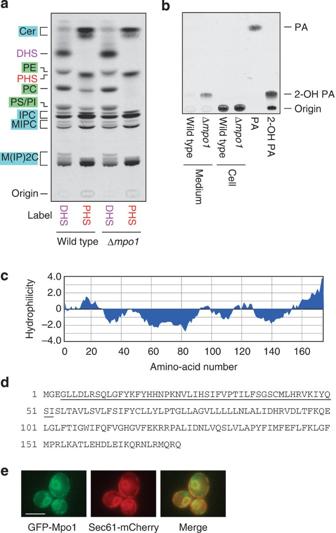Figure 5:MPO1is involved in PHS-to-glycerophospholipid metabolism. (a,b) BY4741 (wild-type) and 4378 (Δmpo1) cells were incubated with 0.1 μCi [3H]DHS/[3H]PHS at 30 °C for 3 h. Lipids were extracted from the cells (a,b) and cell culture medium (b), separated by normal-phase TLC with chloroform/methanol/4.2 N ammonia (9:7:2, v/v) (a) and hexane/diethyl ether/acetic acid (30:70:1, v/v) (b), and detected by autoradiography. PA, palmitic acid; 2-OH PA, 2-hydroxypalmitic acid. (c) A hydrophilicity plot of the Mpo1 protein was generated using MacVector software (MacVector Inc) with Kyte and Doolittle hydrophilicity values44(window size of 15). (d) Amino-acid sequence of the Mpo1 protein. The underlined region shares a weak sequence similarity with the NAD+-binding domain of Sir2. (e) YOY158 (SEC61-mCherry) cells bearing a pNK47 (GFP-MPO1) plasmid were grown in SC medium lacking uracil at 30 °C. Expression of GFP-Mpo1 was induced by transferring cells to SC medium lacking uracil and methionine for 30 min. Cells were analyzed by fluorescence microscopy using a DM5000B fluorescence microscope (Leica Microsystems). Scale bar, 5 μm. Figure 5: MPO1 is involved in PHS-to-glycerophospholipid metabolism. ( a , b ) BY4741 (wild-type) and 4378 (Δ mpo1 ) cells were incubated with 0.1 μCi [ 3 H]DHS/[ 3 H]PHS at 30 °C for 3 h. Lipids were extracted from the cells ( a , b ) and cell culture medium ( b ), separated by normal-phase TLC with chloroform/methanol/4.2 N ammonia (9:7:2, v/v) ( a ) and hexane/diethyl ether/acetic acid (30:70:1, v/v) ( b ), and detected by autoradiography. PA, palmitic acid; 2-OH PA, 2-hydroxypalmitic acid. ( c ) A hydrophilicity plot of the Mpo1 protein was generated using MacVector software (MacVector Inc) with Kyte and Doolittle hydrophilicity values [44] (window size of 15). ( d ) Amino-acid sequence of the Mpo1 protein. The underlined region shares a weak sequence similarity with the NAD + -binding domain of Sir2. ( e ) YOY158 ( SEC61-mCherry ) cells bearing a pNK47 ( GFP-MPO1 ) plasmid were grown in SC medium lacking uracil at 30 °C. Expression of GFP-Mpo1 was induced by transferring cells to SC medium lacking uracil and methionine for 30 min. Cells were analyzed by fluorescence microscopy using a DM5000B fluorescence microscope (Leica Microsystems). Scale bar, 5 μm. Full size image Mpo1 belongs to the DUF962 (DUF) superfamily ( http://www.ebi.ac.uk/interpro/entry/IPR009305 ). To date, over 3,000 proteins from bacteria, fungi, plants and protists have been registered as DUF962 family members. However, no functions have been reported for any of these members. Mpo1 is a relatively small protein, and its predicted molecular mass is 20.2 kDa. It is also a highly hydrophobic protein and may possess two to four transmembrane segments ( Fig. 5c,d ). Mpo1 contains no apparent domain or sequence motif found in other protein families. However, the N-terminal region of Mpo1 ( Fig. 5d , underlined) shares weak sequence similarity with the NAD + -binding domain of the histone deacetylase Sir2, implying that Mpo1 may function as an oxidase with NAD + acting as the oxidant. We confirmed the ER localization of Mpo1 using N-terminally GFP-tagged Mpo1 protein. GFP-Mpo1 exhibited a typical ER pattern, that is, two-ring structures of nuclear ER that surround the nucleus, and cortical ERs ( Fig. 5e ). GFP-Mpo1 indeed co-localized with the mCherry-tagged ER marker Sec61. PHS is metabolized to odd-numbered FAs in mammalian cells We next examined the metabolism of PHS in mammalian cells using CHO-K1 cells via a [ 3 H]PHS-labelling experiment. Comparing the metabolism of PHS with that of DHS, sphingomyelin slightly decreased, whereas monohexosylceramide increased ( Fig. 6a ; see Supplementary Fig. 6 for the sphingolipid biosynthetic pathway in mammals). Glycerophospholipid levels appeared to be equivalent between [ 3 H]DHS- and [ 3 H]PHS-labelling experiments, in contrast to the case of yeast. To examine the FA species derived from PHS in mammals, PHS metabolites were analyzed by reverse-phase TLC after methyl-esterification. We observed production of C15:0 FAME and, to a lesser extent, its elongated product C17:0 FAME, both of which were resistant to KIO 4 /KMnO 4 treatment ( Fig. 6b ). By [ 3 H]DHS labelling, C16:0 FAME and its elongated product C18:0 FAME were generated ( Fig. 6b ). Similar results were obtained when human embryonic kidney (HEK) 293T cells were subjected to the analyses ( Fig. 6c,d ). Thus, although PHS was metabolized to odd-numbered FAs in mammalian cells as well as in yeast, the odd-numbered FAs generated in yeast were partly desaturated, whereas mammals produced elongated odd-numbered FAs. 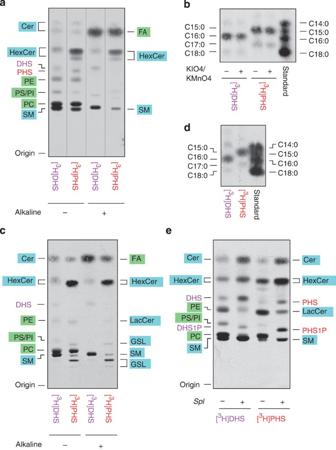Figure 6: PHS is metabolized to odd-numbered FAs in mammals. (a–e) CHO-K1 (a,b), HEK 293T (c,d) and mouse embryonic carcinoma F9 (Spl+/+) and F9-2 (Spl−/−) cells (e) were labelled with 0.1 μCi (2.25 nmol) [3H]DHS or [3H]PHS at 30 °C for 5 h. (a,c,e) Lipids were extracted, treated with or without alkaline solution and separated by normal-phase TLC with 1-butanol/acetic acid/water (3:1:1, v/v). GSL, glycosphingolipid; HexCer, monohexosylceramide; LacCer, lactosylceramide; SM, sphingomyelin. (b,d) Lipids were extracted and treated with alkaline solution. The released FAs were methyl-esterified, and the resulting FAMEs were incubated with or without KMnO4/KIO4solution, extracted with hexane and separated by reverse-phase TLC with chloroform/methanol/water (5:15:1, v/v). The standard containing C14:0, C15:0, C16:0 and C18:0-FAMEs was a mixture of FA elongation products prepared as inSupplementary Fig. 1. Figure 6: PHS is metabolized to odd-numbered FAs in mammals. ( a – e ) CHO-K1 ( a , b ), HEK 293T ( c , d ) and mouse embryonic carcinoma F9 ( Spl +/+ ) and F9-2 ( Spl −/− ) cells ( e ) were labelled with 0.1 μCi (2.25 nmol) [ 3 H]DHS or [ 3 H]PHS at 30 °C for 5 h. ( a , c , e ) Lipids were extracted, treated with or without alkaline solution and separated by normal-phase TLC with 1-butanol/acetic acid/water (3:1:1, v/v). GSL, glycosphingolipid; HexCer, monohexosylceramide; LacCer, lactosylceramide; SM, sphingomyelin. ( b , d ) Lipids were extracted and treated with alkaline solution. The released FAs were methyl-esterified, and the resulting FAMEs were incubated with or without KMnO 4 /KIO 4 solution, extracted with hexane and separated by reverse-phase TLC with chloroform/methanol/water (5:15:1, v/v). The standard containing C14:0, C15:0, C16:0 and C18:0-FAMEs was a mixture of FA elongation products prepared as in Supplementary Fig. 1 . Full size image In yeast, PHS was metabolized to glycerophospholipids after conversion to PHS1P and cleavage by LCBP/S1P lyase. To investigate whether PHS is also metabolized via a similar pathway in mammals, we performed the [ 3 H]DHS- and [ 3 H]PHS-labelling experiments with mouse embryonic carcinoma F9 cells and its mutant cell line (S1P lyase Spl gene (the DPL1 homologue)-deficient; Fig. 6e ). Consistent with our previous results [17] , the metabolism of DHS to glycerophospholipids was almost completely abolished in F9 Spl −/− cells. Similarly, the metabolism of PHS to glycerophospholipids was also impaired in F9 Spl −/− cells. Thus, the metabolism of PHS to glycerophospholipids is dependent on S1P lyase in mammalian cells as well as in yeast. In the present study, we demonstrate for the first time that PHS is metabolized to glycerophospholipids in both yeast and mammalian cells ( Figs 1d and 6a,c,e ), as are other LCBs including sphingosine and DHS [17] . Although sphingosine and DHS were metabolized to palmitic acid (C16:0) and its desaturated (C16:1) or elongated (C18:0) derivative in glycerophospholipids, PHS was converted to odd-numbered pentadecanoic acid (C15:0) and its derivatives (C15:1, C17:0 and 17:1; Figs 2 and 6 ). The existence of odd-numbered FAs in mammals has been known since the 1950s (refs 30 , 31 ). However, their origin remains unclear, although dietary intake and de novo FA synthesis by FA synthase using propionyl-CoA have been considered to be sources of odd-numbered FAs [3] , [32] , [33] . FA synthase normally utilizes acetyl-acyl carrier protein (ACP) as a starting material for condensation with malonyl-ACP, producing even-numbered FAs, mainly palmitic acid. However, a small fraction of propionyl-CoA produced during amino acid and cholesterol metabolism appears to be converted to propionyl-ACP, which is then used for FA synthesis. When mice were fed tripropionin, levels of odd-numbered FAs were increased in depot fat [32] . In addition, propionic acidemia patients, who cannot metabolize propionyl-CoA because of a defect in propionyl-CoA decarboxylase, were found to have approximately four- to fivefold higher levels of odd-numbered FAs in their erythrocytes, plasma, liver and subcutaneous tissue compared with controls [3] . However, the contribution of the propionate-derived odd-numbered FAs relative to total odd-numbered FAs under normal conditions and other tissues remains unknown. Here we report that PHS was the major source of odd-numbered FAs, at least in yeast ( Fig. 2c,d and Supplementary Fig. 2 ). In mammals, PHS is localized to specific tissues such as the skin and the small intestine [7] , [12] , [13] , [14] . Consistent with the abundance of PHS in the skin, odd-numbered Cers also exist in the skin at extremely high levels [4] , suggesting that PHS may be the major source of odd-numbered FAs in PHS-rich mammalian tissues. We observed that the metabolism of PHS to glycerophospholipids depended on the LCB kinase Lcb4, LCBP lyase Dpl1, fatty aldehyde dehydrogenase Hfd1 and acyl-CoA synthetases Faa1 and Faa4 ( Fig. 4a ). Therefore, PHS is first converted to PHS1P by Lcb4 and degraded to 2-hydroxyhexadecanal by Dpl1 ( Fig. 7 ). This degradation step is the key determinant of the metabolic flow of LCB/LCBP ( Fig. 3 ). 2-Hydroxyhexadecanal is then oxidized to 2-hydroxypalmitic acid by Hfd1 ( Fig. 7 ). We detected 2-hydroxypalmitic acid and pentadecanoic acid in the medium of Δ faa1 Δ faa4 cells ( Fig. 4b ), suggesting that both 2-hydroxypalmitic acid and pentadecanoic acid are substrates of the acyl-CoA synthetases Faa1 and Faa4 in the PHS metabolic pathway. Thus, the Hfd1 product 2-hydroxypalmitic acid may be converted to 2-hydroxypalmitoyl-CoA by Faa1 and Faa4 in the next step ( Fig. 7 ). Although the exact role of Mpo1 is unclear at present, Mpo1 must be involved in a PHS-specific reaction, that is, a reaction that is not involved in DHS metabolism ( Fig. 5a ). Given that Mpo1 is a putative NAD + -binding protein, we hypothesize that Mpo1 may be involved in the α-oxidation of 2-hydroxypalmitoyl-CoA, producing pentadecanoic acid or other metabolites such as pentadecanal that can be metabolized to pentadecanoic acid. Pentadecanoic acid is finally converted to pentadecanoyl-CoA by Faa1 and Faa4 for glycerophospholipid synthesis ( Fig. 7 ). The observation that pentadecanoic acid was detected in the medium of Δ faa1 Δ faa4 cells ( Fig. 4b ) suggests that metabolism of at least some 2-hydroxypalmitic acid can still proceed to pentadecanoic acid even in the absence of Faa1 and Faa4. Yeast contains seven acyl-CoA synthetases (Faa1, Faa2, Faa3, Faa4, Fat1, Fat2 and Acs1). Therefore, acyl-CoA synthetases other than Faa1 and Faa4 may have residual activity towards 2-hydroxypalmitic acid in Δ faa1 Δ faa4 cells. As 2-hydroxypalmitic acid was detected in the medium of Δ mpo1 cells ( Fig. 5b ), we speculate that 2-hydroxypalmitoyl-CoA is converted to 2-hydroxypalmitic acid by an acyl-CoA hydrolase and is released into the medium in the Δ mpo1 cells. 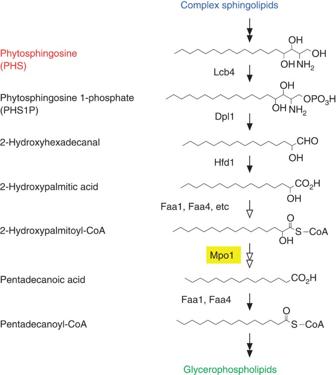Figure 7: Proposed metabolic pathway of PHS to pentadecanoyl-CoA. The proposed pathway and enzymes responsible for PHS metabolism in yeast are shown. PHS is first phosphorylated by LCBP kinase Lcb4. The resulting PHS1P is cleaved to 2-hydroxyhexadecanal by LCBP lyase Dpl1. The fatty aldehyde dehydrogenase Hfd1 oxidizes 2-hydroxyhexadecanal to 2-hydroxypalmitic acid. Faa1, Faa4 and probably other acyl-CoA synthetases may catalyze conversion of 2-hydroxypalmitic acid to 2-hydroxypalmitoyl-CoA. Mpo1 may convert 2-hydroxypalmitoyl-CoA to pentadecanoic acid or another metabolite leading to pentadecanoic acid. Finally, pentadecanoic acid is activated to pentadecanoyl-CoA by the acyl-CoA synthetases Faa1 and Faa4 and incorporated into glycerophospholipids. Open arrows represent reactions that are yet to be fully elucidated. Figure 7: Proposed metabolic pathway of PHS to pentadecanoyl-CoA. The proposed pathway and enzymes responsible for PHS metabolism in yeast are shown. PHS is first phosphorylated by LCBP kinase Lcb4. The resulting PHS1P is cleaved to 2-hydroxyhexadecanal by LCBP lyase Dpl1. The fatty aldehyde dehydrogenase Hfd1 oxidizes 2-hydroxyhexadecanal to 2-hydroxypalmitic acid. Faa1, Faa4 and probably other acyl-CoA synthetases may catalyze conversion of 2-hydroxypalmitic acid to 2-hydroxypalmitoyl-CoA. Mpo1 may convert 2-hydroxypalmitoyl-CoA to pentadecanoic acid or another metabolite leading to pentadecanoic acid. Finally, pentadecanoic acid is activated to pentadecanoyl-CoA by the acyl-CoA synthetases Faa1 and Faa4 and incorporated into glycerophospholipids. Open arrows represent reactions that are yet to be fully elucidated. Full size image Although peroxisomes are known to be involved in α-oxidation [34] , we found that Mpo1 was localized to the ER ( Fig. 5e ), similar to other enzymes involved in LCBP metabolism [16] . We examined the involvement of peroxisomes in PHS metabolism by using yeast deletion mutants for the peroxisomal translocation machinery PEX2 and PEX12 and the ABC transporter subunits PXA1 and PXA2 that are required for importing long-chain FA into peroxisomes. However, PHS was metabolized as normal in these mutants ( Supplementary Fig. 7 ). Thus, our results suggest that peroxisomes are unlikely to be involved in the PHS metabolism; instead, all reactions in the PHS metabolic pathway are likely to occur in the ER. Mpo1 belongs to the large protein family DUF962, whose functions are unknown at present. Our findings suggest that Mpo1 is involved in the α-oxidation of 2-hydroxyacyl-CoAs. As the function of the DUF962 family has been elucidated here, we will refer to it as the Mpo1 family hereafter. Mpo1 family members exist in bacteria, fungi, plants and protists; 2-hydroxy FAs also exist in these organisms [20] , although its presence in protists has not been examined. It is therefore highly likely that Mpo1 family members are involved in the α-oxidation of 2-hydroxyacyl-CoAs in general. Our results indicate that PHS is metabolized to odd-numbered FAs in mammals ( Fig. 6 ). However, Mpo1 family members are not expressed in mammals, in contrast to other LCB/LCBP metabolic enzymes conserved between yeast and mammals [16] . PHS seems to have once disappeared in the course of evolution, when Animalia diverged from Plantae. Therefore, members of lower Animalia do not possess PHS. However, mammals again evolutionarily acquired the ability to produce PHS, likely due to the requirement for PHS to fulfill the functions in specific tissues. We speculate that Mpo1 homologues were lost at the same time as when PHS disappeared in Animalia. Instead, mammals may have independently evolved an α-oxidase from other protein families, when they began to utilize PHS. LCBs have two hydroxyl groups and one amino group in common, both of which can form hydrogen bonds. As PHS contains an additional hydroxyl group, PHS may possess different properties compared with other LCBs and specific functions by interacting with other lipids or proteins with higher affinity because of additional hydrogen bond formation. Therefore, PHS may be important for PHS-containing tissues such as the skin and small intestine, and its reduction may lead to disorders. Indeed, a decrease in PHS-containing Cer levels has been observed in psoriatic scale [35] . In addition, the degradation pathway must also be important for the maintenance of appropriate levels of PHS, as it is for other biomolecules in general. Indeed, several metabolic disorders, including sphingolipidoses [36] , are known to be due to defects in certain lipid degradation pathway. The PHS metabolite, odd-numbered FAs, is much less common than even-numbered FAs, and both are similarly metabolized to glycerophospholipids. Thus, odd-numbered FA itself might not have physiological significance. However, the PHS metabolic pathway that we have elucidated here may be important for the maintenance of cellular PHS levels and clearance of PHS metabolites such as 2-hydroxy FAs, and disorders can arise from its deregulation. Both PHS and 2-hydroxypalmitic acid are incorporated into sphingolipids only, and are not used in other lipids. In addition, they cannot to be subjected to β-oxidation in their current forms. The PHS metabolic pathway revealed here converts them to the metabolizable compound, non-hydroxylated pentadecanoic acid. Pentadecanoic acid can undergo desaturation, elongation, incorporation into glycerophospholipids and mitochondrial β-oxidation, where the final round product propionyl-CoA is converted to succinyl-CoA and subsequently metabolized in the citric acid cycle [37] . In mammals, there remain a large number of orphan G protein-coupled receptors. Recent developments in lipidomics analysis have led to the discovery of many novel lipid metabolites, some of which have been determined to be ligands of orphan G protein-coupled receptors. Our elucidation of the PHS metabolic pathway encourages the search for novel bioactive lipid molecules in the derivatives of PHS metabolites. Yeast strains and media The Saccharomyces cerevisiae strains used in this study are listed in Supplementary Table 1 . BY4741 cells [38] were obtained from Open Biosystems. Chromosome fusion of mCherry to the 3′-terminus of the SEC61 gene was performed using PCR-based gene disruption and modification [39] . Cells were grown in YPD medium (1% yeast extract, 2% peptone and 2% D -glucose), synthetic complete (SC) medium (0.67% yeast nitrogen base, 2% D -glucose, 20 mg l −1 adenine, 20 mg l −1 uracil and an amino-acid mixture) or SC medium lacking uracil (SC-URA; 0.67% yeast nitrogen base, 2% D -glucose, 20 mg l −1 adenine, 20 mg l −1 tryptophan and 0.5% casamino acids). Cell culture HEK 293T (American Type Culture Collection (ATCC); cat. no. CRL-3216) and mouse embryonic carcinoma and F9 cells (ATCC; CRL-1720) were grown in Dulbecco’s modified Eagle’s medium (Sigma/Sigma-Aldrich), whereas Chinese hamster ovary CHO-K1 cells (ATCC; CRL-9618) were cultured in Ham’s F-12 medium (Sigma). Each medium contained 10% fetal bovine serum, 100 U ml −1 penicillin and 100 μg ml −1 streptomycin. HEK 293T and F9 cells were grown in dishes coated with 0.3% collagen and 0.1% gelatin, respectively. Spl -deficient F9 cells (F9-2) have been described previously [40] . Plasmids The pAKNF316 plasmid ( URA3 marker) is a yeast expression vector and was designed to produce an N-terminal 3xFLAG-tagged protein under the control of the GAPDH ( TDH3 ) promoter. The pAN9 ( 3xFLAG-DPL1 ) and pAN13 ( 3xFLAG-LCB3 ) plasmids were constructed by cloning of DPL1 and LCB3 genes into the pAKNF316 plasmid, respectively. The pTS229 plasmid ( TRP1 marker) encodes 3xFLAG-LCB4 under the control of the GAPDH promoter. The pUG36 plasmid ( URA3 marker), a yeast expression vector constructed to produce a fusion protein with an N-terminal enhanced GFP under the control of the MET15 promoter, was a gift from J. H. Hegemann. The pNK47 ( GFP-MPO1 ) plasmid was constructed by cloning the MPO1 gene into the pUG36 plasmid. Preparation of [11, 12- 3 H]PHS BY4741 cells (100 ml) grown in YPD medium to log phase were labelled at 30 °C for 4 h with 1 mCi [9,10- 3 H]palmitic acid (40 Ci mmol −1 , 10 mCi ml −1 ; American Radiolabeled Chemical). Lipids were extracted and hydrolyzed by HCl/methanol as described elsewhere [41] . Lipids suspended in 300 μl chloroform/methanol (2:1, v/v) were resolved by normal-phase TLC on Silica Gel 60 high-performance TLC plates (Merck) with chloroform/methanol/4.2 N ammonia (9:7:2, v/v) so the leading edge was positioned 2.5 cm from the top. Plates were then dried and resolved with 1-butanol/acetic acid/water (3:1:1, v/v) to the top. PHS was scraped from the TLC plate and was extracted three times using 200 μl ethanol. Silica gel was removed by centrifugation, and the collected lipids were combined. The obtained PHS was estimated to be 0.025 μCi μl −1 by measuring its radioactivity using a liquid scintillation counter (LSC-3600; Aloka) and to be 0.55 mM by comparing its ninhydrin-stained density with cold PHS standard (Enzo Life Sciences). To phosphorylate [11, 12- 3 H]PHS, 8 nCi of [11, 12- 3 H]PHS was incubated with 250 ng of 3xFLAG-Lcb4 for 1 h at 37 °C in 50 μl of buffer A (50 mM HEPES-NaOH (pH 7.5), 150 mM NaCl, 200 mM sorbitol, 1 × Complete protease inhibitor mixture (EDTA-free; Roche Diagnostics), 1 mM phenylmethylsulfonyl fluoride, 1 mM dithiothreitol, 5 mM ATP and 10 mM MgCl 2 ) containing 0.5 mg ml −1 of FA-free BSA (A6003; Sigma). Soluble, non-palmitoylated 3xFLAG-Lcb4 was purified as described previously [42] , by subjecting the soluble fraction prepared from the palmitoyltransferase mutant KHY543 (Δ akr1 ) cells harbouring the pTS229 ( 3xFLAG-LCB4 ) plasmid to incubate with anti-FLAG M2 agarose (Sigma), followed by extensive washing and elution with buffer containing 100 μg ml −1 of 3xFLAG peptide. Lipids were extracted by successive addition and mixing of 187.5 μl of chloroform/methanol/HCl (100:200:1, v/v), 62.5 μl of chloroform and 62.5 μl of 1% KCl. Phases were separated by centrifugation, and the organic phase was recovered, dried and suspended in chloroform/methanol (2:1, v/v). The labelled lipids were resolved by normal-phase TLC on Silica Gel 60 high-performance TLC plates with chloroform/methanol/4.2 N ammonia (9:7:2, v/v). [ 3 H]LCB-labelling assay To prepare [4,5- 3 H]DHS with its radioactivity and concentration identical to [11,12- 3 H]PHS (0.025 μCi μl −1 , 0.55 mM), [4,5- 3 H]DHS (50 Ci mmol −1 ; American Radiolabeled Chemicals) was mixed with cold DHS (Enzo Life Sciences). The [ 3 H]LCB-labelling assay using mammalian cells was performed as described previously [17] , [19] . The [ 3 H]LCB-labelling assay using yeast was conducted as follows. Yeast cells were grown to ~5 × 10 6 cells per ml in YPD medium and then 0.75 ml of cells were labelled with [11,12- 3 H]PHS or [4,5- 3 H]DHS (0.1 μCi (2.2 nmol) or 0.2 μCi (0.44 nmol) as indicated in figure legends) at 30 °C for 3 h. After labelling, the cells and medium were separated by centrifugation (2,000 g , room temperature, 2 min). Cells were washed with 0.5 ml water and resuspended in 200 μl ethanol/water/diethyl ether/pyridine/15 N ammonia (15:15:5:1:0.018, v/v). After a 15-min incubation at 60 °C with mixing every 5 min, extracted lipids were recovered in the supernatant after centrifugation (8,000 g , room temperature, 1 min). Radioactivity was measured using the liquid scintillation system LSC-3600, and lipid extracts of equal radioactivity were dried. Lipids from the medium were extracted by mixing with successive additions of 3.75 volumes of chloroform/methanol/HCl (100:200:1, v/v), 1.25 volumes of chloroform and 1.25 volumes of 1% KCl. Phases were then separated by centrifugation (8,000 g , room temperature, 1 min), and the organic phase was recovered and dried. Lipids were resuspended in 20 μl chloroform/methanol/water (5:4:1, v/v) and separated by normal-phase TLC on Silica Gel 60 high-performance TLC plates with chloroform/methanol/4.2 N ammonia (9:7:2, v/v) or hexane/diethyl ether/acetic acid (30:70:1, v/v) as the solvent. Note that other than FAs, no labelled lipids were moved from the origin by the latter, highly nonpolar, resolving buffer. Lipids were visualized by spraying the TLC plates with a fluorographic reagent (2.8 mg ml −1 of 2,5-diphenyl-oxazole in 2-methylnaphthalene/1-buthanol (1:3.3, v/v)) and exposing them to X-ray film at −80 °C. The identities of the lipid bands on TLCs have been described previously [17] . Methyl-esterification of FAs, double-bond cleavage assays using KMnO 4 and KIO 4 , and separation of FAMEs by reverse-phase TLC were performed as follows. Lipids extracted from labelled cells with ethanol/water/diethyl ether/pyridine/15 N ammonia (15:15:5:1:0.018, v/v) as described above were treated with 0.25 volumes of 0.5 M NaOH in methanol and incubated at 37 °C for 30 min to liberate the FAs from glycerophospholipids. After neutralization with acetic acid, lipids were extracted by mixing with successive additions of 2.25 volumes of chloroform/methanol (7:11, v/v), 0.94 volumes of chloroform and 0.94 volumes of 1% KCl. Phases were then separated by centrifugation (8,000 g , room temperature, 1 min), and the organic phase was recovered and dried. Lipids were resuspended in 50 μl of chloroform/methanol (2:1, v/v) and separated by normal-phase TLC on Silica Gel 60 high-performance TLC plates with chloroform/methanol/4.2 N ammonia (9:7:2, v/v). FAs were eluted from the silica with ethanol and dried. The prepared FAs or lipids extracted from the medium as described above were methyl-esterified by resuspending the dried lipids in 200 μl of 1 M methanolic HCl and 5% 2,2-dimethoxypropane, followed by incubation at 100 °C for 1 h. Generated FAMEs were extracted from the methanol phase with 300 μl hexane twice, dried and separated by reverse-phase TLC or subjected to double-bond cleavage assays. For the double-bond cleavage assay, lipids were resuspended in 100 μl of 90% acetic acid and divided into two portions of 50 μl each. Lipids were treated with 75 μl of 0.5% KMnO 4 and 0.5% KIO 4 (or 75 μl water for the control) at 37 °C for 1 h, reduced with 15 μl of 20% sodium bisulfite (or 15 μl water for the control) and neutralized with 50 μl of 15 M ammonia. Lipids were then extracted by adding 250 μl chloroform. After phase separation by centrifugation (8,000 g , room temperature, 1 min), the organic phase was recovered and dried. Lipids were resuspended in 20 μl chloroform and separated by reverse-phase TLC on a Silica gel 60 RP-18F 254 s TLC plates (Merck) with chloroform/methanol/water (5:15:1, v/v). Preparation of 32 P-labelled LCBPs Cold DHS and PHS were purchased from Enzo Life Sciences and dissolved in ethanol. The 32 P-labelled LCBPs were prepared by incubating 30 μM LCBs complexed with 0.4 mg ml −1 of FA-free BSA with 13 μCi [γ- 32 P]ATP (3,000 Ci mmol −1 ; Perkin Elmer Life Sciences) and 62.5 ng purified 3xFLAG-Lcb4 (ref. 42 ) at 37 °C for 1 h in 100 μl of buffer B (50 mM HEPES-NaOH (pH 7.5), 150 mM NaCl, 10% glycerol, 1 × Complete protease inhibitor mixture, 1 mM phenylmethylsulfonyl fluoride and 1 mM dithiothreitol) containing 5 mM MgCl 2 . Produced LCBPs were extracted by successive additions of 600 μl of chloroform/methanol (1:2, v/v), 7.5 μl of 15 M ammonia, 400 μl of chloroform and 400 μl of 1% KCl, with mixing. Phases were then separated by centrifugation, and the upper, water phase was recovered and mixed with 600 μl of chloroform and 77 μl of 5 M HCl. Phases were separated by centrifugation again, and the lower, organic phase was recovered, dried and dissolved in ethanol. Cold DHS1P (Sigma) and PHS1P (Avanti Polar Lipids) were first dissolved in methanol at 0.5 mM by incubating at 75 °C, followed by sonication. LCBPs were then diluted to 50 μM in buffer B containing 2 mg ml −1 of FA-free BSA and stored at −30 °C. Each 32 P-labelled LCBP prepared as above was mixed with cold LCBP to the desired concentration before use. Preparation of total membrane fractions Approximately 4 × 10 8 yeast cells were suspended in 3.3 ml of buffer C (100 mM Tris-HCl (pH 9.4) and 40 mM 2-mercaptoethanol), and incubated at room temperature for 10 min. After centrifugation, cells were resuspended in 6.6 ml of buffer D (50 mM Tris-HCl (pH 7.5) and 1.2 M sorbitol), and incubated at 30 °C for 30 min with 0.33 mg Zymolyase 100T (Seikagaku Corporation). The resulting spheroplasts were washed with 3.3 ml of buffer D, suspended in 0.5 ml of buffer B and lysed by sonication. Cell debris was removed by centrifugation (1,000 g , 4 °C, 3 min), and the supernatant was subjected to centrifugation at 100,000 g at 4 °C for 30 min. The pellet (total membrane fractions) was suspended in 750 μl of buffer B by sonication. In vitro LCBP lyase/phosphatase assay The in vitro LCBP lyase/phosphatase assay was performed by incubation of total membrane fractions with LCBP (25 nCi 32 P-labelled LCBP plus desired concentration of cold LCBP), complexed with FA-free BSA, at 37 °C for 10 min in a 50-μl reaction mixture (50 mM HEPES-NaOH (pH 7.5), 150 mM NaCl, 10% glycerol, 1 × Complete protease inhibitor mixture, 1 mM phenylmethylsulfonyl fluoride, 1 mM dithiothreitol and 250 μM pyridoxal 5′-phosphate). After the reaction, the 7-μl reaction mixture was mixed with 33 μl of chloroform/methanol/water/HCl (100:200:30:1, v/v), and 5 μl of the resultant mixture was spotted on Silica Gel 60 high-performance TLC plates and separated with 1-butanol/acetic acid/water (2:1:1, v/v) as the solvent system. Labelled products were detected and quantified by a bioimaging analyzer BAS-2500 (Fuji Photo Film). Lipid analysis by mass spectrometry The FA composition of PC was determined by ultra-performance liquid chromatography (UPLC) coupled with electrospray ionization tandem quadrupole time-of-flight mass spectroscopy (Xevo G2 QTof; Waters) as follows. Yeast cells were grown in SC medium, and lipids were extracted from ~1.2 × 10 8 cells by incubating cell pellets with ethanol/water/diethyl ether/pyridine/15 N ammonia (15:15:5:1:0.018, v/v) at 60 °C for 15 min in the presence of 1 nmol C12:0 PC (Avanti Polar Lipids) as an internal standard. Extracted lipids were then separated by normal-phase TLC with chloroform/methanol/4.2 N ammonia (9:7:2, v/v), and silica containing PC was scraped from the TLC plate. PC was eluted from silica with chloroform/methanol (1:2, v/v), dried, suspended in methanol, resolved by UPLC on a reverse-phase column (AQUITY UPLC BEH C18 column, length 150 mm; Waters) at 45 °C, and detected by mass spectrometry (MS). The flow rate was 0.1 ml min −1 in the binary gradient system using mobile phase A (acetonitrile/water/methanol (4:4:2, v/v) containing 0.1% formic acid and 0.025% ammonia) and mobile phase B (2-propanol/methanol (4:1, v/v) containing 0.1% formic acid and 0.025% ammonia). The elution gradient steps were as follows: 0–10 min, 5% B; 10–50 min, gradient to 80% B; 50–55 min, gradient to 100% B; 55–65 min, 100% B; 65–66 min, gradient to 5% B; 66–80 min, 5% B. The electrospray ionization (ESI) capillary voltage was set at 2.6 kV, sampling cone was at 35 V and extraction cone was at 4 V in negative ion mode. The mass range was set at m/z =500–900, and scan duration was set at 1 s. To discriminate PC species having the same molecular mass but different FA compositions, the same samples used in the above MS analysis were also subjected to MS analysis in MS/MS mode. The m/z ([M+HCOO] − ) of specific PC species, as listed in Supplementary Table 2 , was selected at Q1 ( Supplementary Fig. 8 ), and their FA compositions were determined by analyzing their fragment ions ( Supplementary Table 3 and Supplementary Fig. 9 ). Argon gas was used as the collision gas, and collision energy was set at 30 V. Data analysis and quantification were performed using MassLynx software (Waters). For quantification, levels of PC species with the same molecular mass were first determined by comparing their ion intensities with those of the internal standards in the first MS analyses, and levels of each PC species having specific FA composition were then calculated by comparing the ion intensities of their fragments in the MS/MS analysis. Immunoblotting Immunoblotting was performed as described previously [43] . Proteins were electrotransferred to an Immobilon PVDF membrane (Millipore), which was incubated with primary anti-FLAG M2 antibody (1 μg ml −1 ; Stratagene, Agilent Technologies) for 1 h and then with secondary HRP-conjugated anti-mouse IgG F(ab′) 2 fragment antibody (1:7,500 dilution; GE Healthcare Life Sciences) for an additional 1 h. Labelling was detected using Pierce ECL Western Blotting Substrate (Thermo Fisher Scientific). How to cite this article : Kondo, N. et al. Identification of the phytosphingosine metabolic pathway leading to odd-numbered fatty acids. Nat. Commun. 5:5338 doi: 10.1038/ncomms6338 (2014).